Robust electron pairing in the integer quantum hall effect regime Electron pairing is a rare phenomenon appearing only in a few unique physical systems; for example, superconductors and Kondo-correlated quantum dots. Here, we report on an unexpected electron pairing in the integer quantum Hall effect regime. The pairing takes place within an interfering edge channel in an electronic Fabry–Perot interferometer at a wide range of bulk filling factors, between 2 and 5. We report on three main observations: high-visibility Aharonov–Bohm conductance oscillations with magnetic flux periodicity equal to half the magnetic flux quantum; an interfering quasiparticle charge equal to twice the elementary electron charge as revealed by quantum shot noise measurements, and full dephasing of the pairs' interference by induced dephasing of the adjacent inner edge channel—a manifestation of inter-channel entanglement. Although this pairing phenomenon clearly results from inter-channel interaction, the exact mechanism that leads to electron–electron attraction within a single edge channel is not clear. We believe that substantial efforts are needed in order to clarify these intriguing and unexpected findings. The Fabry–Perot interferometer (FPI) is one of several interferometers implemented in optical [1] , [2] as well as in electronic systems [3] , [4] , [5] , [6] , [7] . Its electronic version [6] , [7] is an excellent platform to demonstrate the wave-particle duality of electrons: interference [4] —a manifestation of wave-like behaviour—alongside with current-fluctuation [8] due to particles discreteness. Moreover, the electronic version of the FPI harbours an exceedingly more complex behaviour due to the interacting nature of electrons. Two distinct regimes of the FPI operating in the QHE regimes have been observed [6] , [7] and theoretically studied [9] , [10] , [11] , [12] : the coherent Aharonov–Bohm (AB) regime, where interactions were thought to play only a minor role and the Coulomb-dominated (CD) regime, where interactions are dominant. In the rather difficult to achieve AB regime, the conductance of the FPI obeys strictly AB interference of independent electrons [13] , [14] , with conductance oscillation phase following ϕ AB =2π AB / φ 0 , where A denotes the area of the interferometer, B the applied magnetic field and φ 0 = h / e =41 μm 2 G the magnetic flux-quantum with h the Planck constant and e the electron charge. Alternatively, in the CD regime, conductance oscillation is due to periodic charging (and discharging) of the FPI with single electrons. Noting that the AB regime is highly desirable as it had been proposed to be a sensitive marker to fractional statistics (abelian or non-abelian) of fractionally charged quasiparticles [15] , [16] , [17] , [18] . We address the FPI in the AB regime, which is formed by two quantum point contacts (QPCs) that serve as electronic beam splitters ( Fig. 1a ). A chiral edge channel impinging from the left is transmitted with amplitude , where r 1 ( r r ) and t 1 ( t r ) are the reflection and transmission amplitudes of the left (right) QPC, respectively. Each term in the above sum stands for a different number n of windings that a coherent electron undergoes. 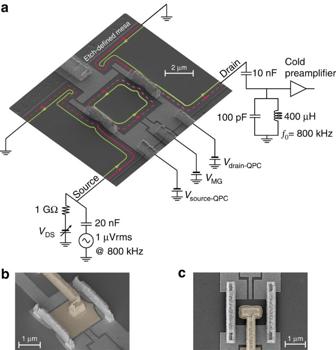Figure 1: Scanning electron microscopy (SEM) images of Fabry–Perot interferometers and the experimental setup. (a) SEM image of a FPI with an illustration of chiral edge channels atνB=2. Edge-channels (green and red lines) run along the interfaces between the mesa (regions with a 2DEG) and regions depleted by etching or gating. The Hall bar is defined by etching and the FPI by gates. Air bridges are used to connect gates and the ohmic contact to the relevant potentials. Partitioned current is denoted by dashed lines. (b) SEM image of a FPI with a (false-coloured) grounded top-gated FPI. (c) SEM image of a FPI with a (false-coloured) grounded centre-ohmic contact. Different FPI sizes were used in the experiments. Hence, the transmission through the interferometer is an oscillating function of the acquired AB phase in a single winding in the FPI: Figure 1: Scanning electron microscopy (SEM) images of Fabry–Perot interferometers and the experimental setup. ( a ) SEM image of a FPI with an illustration of chiral edge channels at ν B =2. Edge-channels (green and red lines) run along the interfaces between the mesa (regions with a 2DEG) and regions depleted by etching or gating. The Hall bar is defined by etching and the FPI by gates. Air bridges are used to connect gates and the ohmic contact to the relevant potentials. Partitioned current is denoted by dashed lines. ( b ) SEM image of a FPI with a (false-coloured) grounded top-gated FPI. ( c ) SEM image of a FPI with a (false-coloured) grounded centre-ohmic contact. Different FPI sizes were used in the experiments. Full size image To first order in the transmission coefficient of the QPCs (namely, ), we have . Evidently, one expects an AB oscillation period in area Δ A = φ 0 / B and in magnetic field Δ B = φ 0 / A . As described in some detail below, the predicted behaviour of equation 1 was precisely observed in a range of bulk filling factors ν B =1–2; however, at fillings around ν B =3–4, the AB periodicity halved, namely, , with , without an observable sign of φ 0 periodicity. Since similar visibilities (contrast, defined as the oscillation amplitude divided by its average), reaching ∼ 60%, were observed in the two filling regimes, interference of only even windings as the cause of the halved periodicity can be excluded. Testing the possibility of electron pairing in the interfering channel, the interfering charge e * was determined by measuring the quantum shot noise, indeed leading to e * ∼ 2 e . These observations were found to be robust and reproducible in FPIs of very different sizes (2–12 μm 2 ), fabricated in different heterostructures (two-dimensional electron gas, 2DEG, density ranged 1.3–2.4 × 10 11 cm −2 ), and at a temperature range 30–130 mK. Moreover, two very different screening methods were employed in order to suppress the CD regime and operate the FPI in the AB regime, both leading to similar results. Measurement setup Our FPIs were realized in a ubiquitous high-mobility 2DEG embedded in AlGaAs-GaAs heterostructure(s), employing optical and E-beam lithography. The FPIs were fabricated as a semi-closed stadium ( Fig. 1 ), terminated with two QPCs; one at the source side and the other at the drain side. A charged modulation gate (MG) allowed varying the FPI’s area. Only the most outer edge channel was partitioned by the QPCs, whereas the impinging inner ones were fully reflected from the QPCs and, likely, the trapped ones circulated inside the FPI. Coulomb interactions were suppressed via two different configurations (illustrated in Fig. 1b,c ), both leading to similar results: the first configuration employs a metallic (Ti-Au) top-gate covering nearly the whole area of the FPI; the second configuration employs a small, grounded, ohmic-contact (alloyed Ni-Ge-Au) in the centre of the incompressible bulk of the FPI. Although the screening process achieved by the grounded ohmic contact is less transparent, it was found to be more effective in suppressing interaction, allowing the fabrication of smaller FPIs operating in the AB regime. This said, the phenomenon reported here is a direct result of inter-edge interactions, while the grounded ohmic contact, as well as the top gate, lower the charging energy of the FPI as a whole (increasing the total self-capacitance) without much effect on the inter-channel capacitance. Differential source-drain conductance was measured by applying an AC voltage of 1 μVrms at 800 kHz; whereas excess quantum shot noise at the drain was measured by driving a variable DC source current, and measuring the noise at a centre frequency of 800 kHz and bandwidth of 10 kHz. For further details see Methods. Conductance measurements The conductance of the FPI was measured as a function of the magnetic flux ϕ , either by varying the magnetic field or the enclosed area (via MG). In the following, we present data taken with two FPIs, each with a centre-ohmic contact, and areas ∼ 2 μm 2 and ∼ 12 μm 2 . 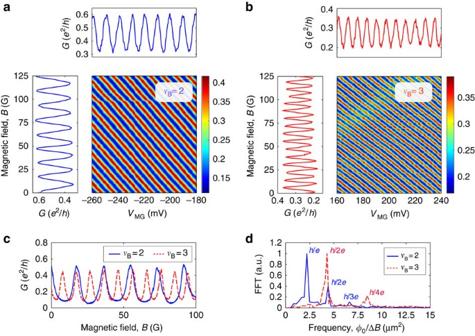Figure 2: Aharonov–Bohm interference in theh/eandh/2eregimes measured with a 2-μm2FPI with grounded centre-ohmic contact. (a,b) ConductanceGof the FPI versus both magnetic fieldBand modulation-gate voltageVMGin theh/eregime (a), and in theh/2eregime (b), qmeasured atB=5.2 T (νB∼2) andB=3 T (νB∼3), respectively. (c) Characteristic AB oscillations with respect to magnetic-fieldBin the two regimes. (d) Corresponding Fourier transforms; noticeably, the second harmonic of theh/eperiodicity coincides with the first harmonic ofh/2eperiodicity. Figure 2 presents the most important data of this work. Starting with the smallest FPI, we plot in Fig. 2a the flux-dependent conductance at ν B ≅ 2 (being representative of similar results in ν B ≅ 1–2.5). Constant phase lines correspond to constant flux; namely, increasing magnetic field necessitates reducing the FPI area. An AB area of 2.1 μm 2 is deduced from Δ B period. However, at ν B ≅ 3 (being a representative of ν B ≅ 2.5–4.5), an unexpected halving of the oscillation periods in B and in V MG is observed ( Fig. 2b ). This is clearly evident in the B dependence oscillations (at constant V MG ) shown in Fig. 2c and their Fourier transform in Fig. 2d . Higher harmonics, corresponding to multiple windings, are also visible in the two regimes. Note an absence of any sign of the fundamental periodicity h / e in the h /2 e regime. Figure 2: Aharonov–Bohm interference in the h / e and h /2 e regimes measured with a 2-μm 2 FPI with grounded centre-ohmic contact. ( a , b ) Conductance G of the FPI versus both magnetic field B and modulation-gate voltage V MG in the h / e regime ( a ), and in the h /2 e regime ( b ), qmeasured at B =5.2 T ( ν B ∼ 2) and B =3 T ( ν B ∼ 3), respectively. ( c ) Characteristic AB oscillations with respect to magnetic-field B in the two regimes. ( d ) Corresponding Fourier transforms; noticeably, the second harmonic of the h / e periodicity coincides with the first harmonic of h /2 e periodicity. Full size image The universality of the results is presented in Fig. 3 , this time with the larger FPI ( A =12.5 μm 2 ), where the dependence of the AB frequencies ( φ 0 /Δ B in Fig. 3a ; 1/Δ V MG in Fig. 3b ) is plotted as a function of bulk filling ν B . In filling ranges ν B <2.5 and ν B >4.5, the normalized oscillation frequency in magnetic field is φ 0 /Δ B e =12 μm 2 —agreeing with FPI area, and is independent of the filling factor. The frequency in MG 1/Δ V MG depends linearly on B , , as expected. This dependence can be easily understood by recalling that the incremental change in charge δ Q is related to δ V MG via the capacitance . Moreover, its relation to the incremental change in area is δ Q=en e δ A , with n e the carrier density. Hence, where e * is the interfering quasiparticle charge in the most outer channel, being in this filling range e . However, in the filling range ν B =3–4.5, the B -dependent normalized frequency is doubled, φ 0 /Δ B 2 e =25 μm 2 , and again independent of filling factor. This doubling suggests halved flux quantum, namely, . Similarly, the AB frequency in 1/Δ V MG has now twice the slope, , again leading to The small deviation from an exact in the region ν B ∼ 2.5–3 ( Fig. 3a,b ) is observed in all the tested samples. The behaviour in the transition region near ν B ∼ 2.5 and ν B ∼ 4.5 is not universal and will not be discussed here. 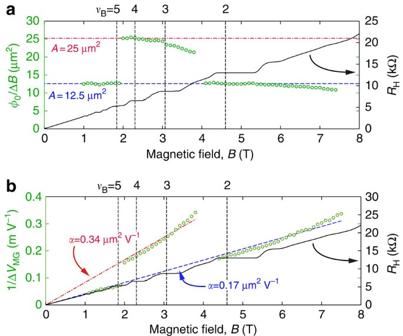Figure 3: Aharonov–Bohm frequency as function of the magnetic field measured with a 12-μm2FPI. (a) Frequency dependence on magnetic field (green, circles) alongside with bulk Hall resistance (black, solid line). (b) Frequency dependence on modulation-gate voltage. In the two graphs, the two dominant frequencies are denoted by blue dashed and red dotted-dashed lines for theh/eandh/2eregimes. The regionsνB<2.5 andνB>4.5 are in agreement with the expected AB oscillations. The frequency in the intermediate region, covering fillingνB=3−4, is doubled in 1/ΔBand has a doubled slope in 1/ΔVMG. This is attributed to a modified magnetic flux quantumφ0*=h/2eand quasi-particle chargee*/e=2. Figure 3: Aharonov–Bohm frequency as function of the magnetic field measured with a 12-μm 2 FPI. ( a ) Frequency dependence on magnetic field (green, circles) alongside with bulk Hall resistance (black, solid line). ( b ) Frequency dependence on modulation-gate voltage. In the two graphs, the two dominant frequencies are denoted by blue dashed and red dotted-dashed lines for the h / e and h /2 e regimes. The regions ν B <2.5 and ν B >4.5 are in agreement with the expected AB oscillations. The frequency in the intermediate region, covering filling ν B =3−4, is doubled in 1/Δ B and has a doubled slope in 1/Δ V MG . This is attributed to a modified magnetic flux quantum φ 0 *= h /2 e and quasi-particle charge e */ e= 2. Full size image Analysis refuting a possibility of even-winding processes Although the doubling of the AB frequencies can be attributed to , with , one can also envision a peculiar preference of only even number of interfering windings, namely, A * =2 A . To distinguish between these two scenarios, we address the visibility of the h /2 e oscillations compared with that of the h / e oscillations. With the visibility of the h / e periodicity in the ∼ 12 μm 2 FPI being ν ( e ,1) max ≈60%, we estimated a dephasing length L γ ≈35 μm (see Supplementary Note 1 ). This value sets an upper-bound for the highest visibility of the second harmonic (two windings in the h / e regime) ν ( e ,2) max ≈10%, which had been confirmed experimentally. However, the highest visibility in the h /2 e regime was found to be ν (2 e ,1) max ≈50%, refuting a peculiar favouring of even number windings. Charge determination via quantum shot noise measurements Shot noise measurements were found to provide an excellent method for a determination of the partitioned charge [19] , [20] , [21] , [22] , [23] , [24] , [25] . For independent and stochastic partitioning events by any scatterer, the expected zero frequency ( hω << eV SD ) excess noise (added noise due to driven current) is given by equation 2, which had been modified to allow e *≠ e (refs 23 , 24 ): where t =| τ | 2 is the transmission coefficient, I the impinging current, T the electron-temperature, V SD source-drain DC-bias and . Noise measurements were first conducted with a single QPC partitioning the outer edge channel at v B =2 and v B =3. A partitioned charge e *= e was extracted in a wide range of transmission coefficients using equation 2 ( Fig. 4a,b ). The FPI was then formed by pinching the second QPC with noise measured in the h / e regime, leading to e *= e ( Fig. 4c , Supplementary Note 2 and Supplementary Fig. 1 ). In the h /2 e regime, on the other hand, the quasiparticle charge was found consistently to be e * ∼ 2 e ( Fig. 4d ). Note that very large Fano factors, defined here as , were found when the visibility was very high, which is attributed to phase noise due to charge fluctuations [26] , [27] , as, when visibility is high, a small variation in the phase might lead to large variation of the transmission. 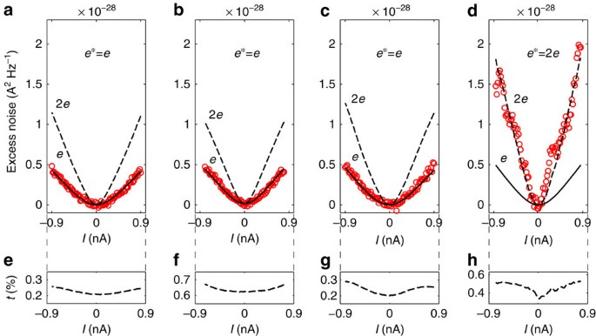Figure 4: Excess shot noise and transmission revealing a quasi-particle charge in the different filling regimes. Measured excess noise (red circles) and expected noise according to equation 2 for quasi-particle chargee*=e(black, solid) and fore*=2e(black, dashed) are plotted ina–das function of source-drain DC currentISD. Lower panels show the conductance as function of source-drain DC currentISD. (a) Excess noise of a single QPC atνB=2; (b) excess noise of a single QPC atνB=3; (c) excess noise of a FPI atνB=2; (d) excess noise of a FPI atνB=3. (e–h) Bias-dependent transmission, given by the ratio of the transmitted current over the incident one, measured for the same devices and setting asa–d, respectively. Figure 4: Excess shot noise and transmission revealing a quasi-particle charge in the different filling regimes. Measured excess noise (red circles) and expected noise according to equation 2 for quasi-particle charge e *= e (black, solid) and for e *=2 e (black, dashed) are plotted in a – d as function of source-drain DC current I SD . Lower panels show the conductance as function of source-drain DC current I SD . ( a ) Excess noise of a single QPC at ν B =2; ( b ) excess noise of a single QPC at ν B =3; ( c ) excess noise of a FPI at ν B =2; ( d ) excess noise of a FPI at ν B =3. ( e–h ) Bias-dependent transmission, given by the ratio of the transmitted current over the incident one, measured for the same devices and setting as a – d , respectively. Full size image Inter-edge interaction To test the effect of inter-channel interaction, we modified further the FPI by adding an additional centre-QPC between the edge of the FPI and the centre-ohmic contact (see scanning electron microscopy image in Fig. 5a ). This configuration allows selective reflection of in-bound edge channels to the centre-contact; thus dephasing them and fixing their Fermi energy at ground. Starting at filling ν B =2 with oscillation periodicity h / e , we plotted the transmission of the centre-QPC (to be distinguished from the reflection to the centre-ohmic) and the oscillation visibility of the most outer edge channel as function of the centre-QPC gate voltage ( Fig. 5b ). As expected, the visibility quenches when the interfering edge channel is fully reflected to the centre-ohmic contact. 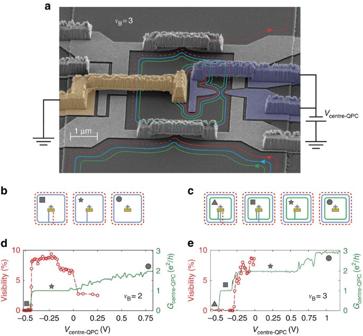Figure 5: The effect of selective reflection of edge channels into the grounded centre-ohmic contact on the visibility. (a) Scanning electron microscopy image of a 12-μm2FPI with a centre-ohmic contact (gold, false-colour) and an additional centre-QPC (blue, false-colour) placed along the FPI edge. An illustration of the edge channels is given forνB∼3 with the most inner edge channel reflected by the centre-QPC into the centre-ohmic contact. ‘Cold’ edges, originating from the ground, are not plotted and dashed lines represent partitioned current. (b,c) Representations of the different configurations distinguished by the number of channels reflected from the FPI’s edge to the centre ohmic contact in theh/eregime (b) and in theh/2eregime (c) measured atνB∼2 andνB∼3, respectively. Circle, star, square and triangle represent zero, one, two and three reflected edges, respectively. (d) ConductanceG(green, solid line) of the centre-QPC plotted alongside with the visibility of the AB oscillations (red, dashed line) atνB=2. The visibility diminishes as the centre-QPC reflects the outer channel to ground. (e) The same measurement as ind, but atνB=3. Surprisingly, here, the visibility fully diminishes once the second channel is reflected to ground. Both indande, the visibility is shown only in the segment of interest, whereas, at higher voltages, the visibility does not vanish, but maintains a relatively constant value. Figure 5: The effect of selective reflection of edge channels into the grounded centre-ohmic contact on the visibility. ( a ) Scanning electron microscopy image of a 12-μm 2 FPI with a centre-ohmic contact (gold, false-colour) and an additional centre-QPC (blue, false-colour) placed along the FPI edge. An illustration of the edge channels is given for ν B ∼ 3 with the most inner edge channel reflected by the centre-QPC into the centre-ohmic contact. ‘Cold’ edges, originating from the ground, are not plotted and dashed lines represent partitioned current. ( b , c ) Representations of the different configurations distinguished by the number of channels reflected from the FPI’s edge to the centre ohmic contact in the h / e regime ( b ) and in the h /2 e regime ( c ) measured at ν B ∼ 2 and ν B ∼ 3, respectively. Circle, star, square and triangle represent zero, one, two and three reflected edges, respectively. ( d ) Conductance G (green, solid line) of the centre-QPC plotted alongside with the visibility of the AB oscillations (red, dashed line) at ν B =2. The visibility diminishes as the centre-QPC reflects the outer channel to ground. ( e ) The same measurement as in d , but at ν B =3. Surprisingly, here, the visibility fully diminishes once the second channel is reflected to ground. Both in d and e , the visibility is shown only in the segment of interest, whereas, at higher voltages, the visibility does not vanish, but maintains a relatively constant value. Full size image Now, in ν B ∼ 3, with oscillation periodicity h /2 e , the behaviour is entirely different. The visibility of the h /2 e periodicity (with all its harmonics) quenches rapidly as soon as the adjacent second edge channel is reflected to the centre-contact—with no sign of interference at all ( Fig. 5c ). We wish to stress that when the h /2 e periodicity quenches, the outer edge channel is uninterruptedly fully transmitted through the centre-QPC. As no tunnelling was observed between these two adjacent edge channels (with an upper limit of 2pA; see Supplementary Note 3 ), this result demonstrates that the coherence of the second edge channel is indispensable for the observation of h /2 e periodicity of the outer edge channel. Employing charge measurement throughout the above-described dephasing process, we plot again in an expanded scale the visibility and the FPI conductance (proportional to the transmission of the outer edge channel) as function of V centre-QPC in Fig. 6a , alongside with the partitioned charge in Fig. 6b . Since the conductance maintains its slope, as the second channel is gradually reflected to ground, it is clear that no current from the outer channel is being lost to the second channel. However, as the coherence of the h /2 e periodicity gradually diminishes, the quasiparticle charge drops gradually from e * ∼ 2 e to e *= e . Noting, that as the transmission of the FPI is highly sensitive to those of the two QPCs and the AB phase, each charge value was determined by averaging the charge measured in a wide span of AB phases at a fixed setting of QPCs. It is hence clear that an interfering charge e * ∼ 2 e is always associated not only with the doubling of the AB frequency, but also with a significant visibility (coherence). 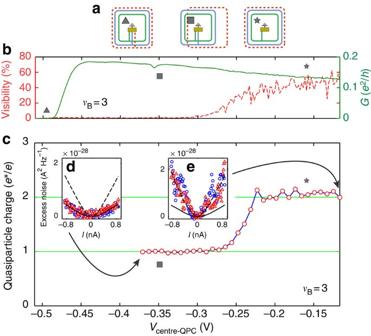Figure 6: The effect of selective reflection of edge channels into the centre-ohmic contact on the quasi-particle charge at theh/2eregime. (a) Representations of the different configurations distinguished by the number of channels reflected from the FPI’s edge to the centre-ohmic contact. Star, square and triangle represent one, two and three reflected edges, respectively. (b) ConductanceGof the FPI (green, solid line) and its visibility (red, dashed line) versus the centre-QPC voltageVcentre-QPC. An expanded scale of the conductance vanishing when the most outer edge channel is reflected to ground at the centre-QPC, whereas the visibility diminishes when the second edge channel is reflected. (c) The quasi-particle charge versusVcentre-QPC. A clear coincidence between the diminishing of the visibility inband the reduction of the charge frome*∼2etoe*=eis found. Insetsd,e: two characteristic noise measurements (red triangles and blue circles) from which charge is extracted and then averaged. The expected noise for the first is plotted according to equation 2 for e*=e (black, solid) ande*=2e(black, dashed). Figure 6: The effect of selective reflection of edge channels into the centre-ohmic contact on the quasi-particle charge at the h /2 e regime. ( a ) Representations of the different configurations distinguished by the number of channels reflected from the FPI’s edge to the centre-ohmic contact. Star, square and triangle represent one, two and three reflected edges, respectively. ( b ) Conductance G of the FPI (green, solid line) and its visibility (red, dashed line) versus the centre-QPC voltage V centre-QPC . An expanded scale of the conductance vanishing when the most outer edge channel is reflected to ground at the centre-QPC, whereas the visibility diminishes when the second edge channel is reflected. ( c ) The quasi-particle charge versus V centre-QPC . A clear coincidence between the diminishing of the visibility in b and the reduction of the charge from e * ∼ 2 e to e *= e is found. Insets d , e : two characteristic noise measurements (red triangles and blue circles) from which charge is extracted and then averaged. The expected noise for the first is plotted according to equation 2 for e*=e (black, solid) and e *=2 e (black, dashed). Full size image Observation of h /2 e periodicity (and higher harmonics) in other electronic systems, such as a CD FPI [6] , [7] and a CD quantum anti-dot [28] , [29] , [30] , have been reported in the past. In these examples, the nonlinear conductance exhibited the ubiquitous Coulomb diamonds [28] , [31] , and the oscillation periodicity with respect to magnetic field scaled inversely with the number of fully transmitted channels through the device [6] , [30] , [32] , [33] , [34] . These two features clearly differ from our observation in the AB–FPI. It may be useful to recapitulate the main results in this work for the interference of the most outer edge channel of the FPI: Although the bare FPI is heavily dominated by Coulomb interactions, thus fully masking the AB interference, our FPI had been modified to suppress the interactions (mostly the intra-channels) and thus showed clear AB behaviour. Two methods were implemented for screening the FPI: a grounded small centre-ohmic contact added to the bulk, and a top-gate covering the device (for more information see Supplementary Notes 4 and 5 and Supplementary Figs 2 and 3 ); different area interferometers, ranging from ∼ 2 to ∼ 12 μm 2 (for more information see Supplementary Note 5 and Supplementary Fig. 4 ), fabricated on different heterostructures, showed qualitatively similar results; the FPIs were tested in a wide range of QPCs transmissions (see Supplementary Note 6 and Supplementary Fig. 5 ); at bulk fillings ν B =1–2.5, the AB periodicity in magnetic field and in MG voltage (affecting the AB area) corresponded to flux periodicity of φ 0 =h / e ; namely, single electron interference. At this range, the interfering charge, determined by shot noise measurement, was e *= e ; at bulk fillings ν B =2.5–4.5, the periodicity in magnetic field and MG voltage halved; namely, with a flux periodicity φ 0 =h /2 e . The interfering charge, measured by shot noise, was e *=2 e ; dephasing the second edge channel (second spin-split Landau level) in filling range ν B =1–2.5 (by shorting the second channel to the centre-ohmic) did not affect the h / e oscillation and the interfering charge; dephasing the second edge channel in filling range ν B =2.5–4.5, fully dephased the h /2 e oscillations and simultaneously lowered the partitioned charge to e *= e ; tunnelling current between adjacent edge channels was not observed (see also Supplementary Note 3 and Supplementary Fig. 6 ); the temperature dependence of the visibility in the h / e and the h /2 e regimes was very similar (see Supplementary Fig. 7 ); decaying exponentially , with T 0 ∼ 25–40 mK; the dependence of the visibility on the transmission of the QPCs was very similar in both regimes (see Supplementary Fig. 8 ); although the transition regions near ν B =2.5 and ν B =4.5 are complex and sample dependent, near ν B =4.5 a coexistence of the two periods, h / e and the h /2 e —being in phase—was observed (see Supplementary Note 7 and Supplementary Fig. 9 ). Moreover, dephasing the h /2 e periodicity did not affect the h / e periodicity (see Supplementary Note 7 and Supplementary Fig. 10 ); allowing the second edge channel to interfere (while the outer channel is fully transmitted), we find only the ubiquitous h / e oscillation in all bulk filling factors (see Supplementary Fig. 8 ). Our results reveal an emergent, and robust, electron pairing in a coherent chiral edge channel, hence, intimately tied to an interfering process. Clear evidence of inter-channel entanglement between the interfering channel and the adjacent one takes place under the pairing conditions. Although Cooper pairing is phonon mediated, here the exact mechanism that leads to intra-channel two-electron attraction is not understood. An important question remains whether the observed phenomenon is general and can be reproduced in other correlated quantum systems. Screening techniques As mentioned in the text, all measurements are performed in the AB -dominated regime, as opposed to the CD regime. The CD regime is avoided by reducing the charging energy of the FPI. This was done by two different techniques, which we detail here further to that discussed in the text. The first, and previously reported [6] , [7] , technique consists of placing a top gate, namely thin layers of 50 Å Ti -150 Å Au on top of the heterostructure, covering the whole area of the FPI, being 73 nm away from the 2DEG. The top gate accommodates image-charge of the charge variations in the 2DEG, and thus induces effective screening and suppression of Coulomb interaction. In other words, the top gate increases the capacitance of the device, and reduces the charging energy of the FPI. Nonetheless, although this technique works well for the bigger FPIs utilized (areas larger than 12 μm 2 ), it does not work for arbitrarily small device. For example, devices of area smaller than 4 μm 2 diameter have been found to be CD, even if covered by top gate [6] , [7] . This was attributed to the different scaling of the capacitances with diameter [10] . The second technique, unreported previously to our knowledge, consists of 106 nm Au/53 nm Ge/40 nm Ni ohmic contacts (OC) alloyed to the heterostructure. Although contacts act normally as sources and drains, here we employ them not for their resistive coupling but for the capacitive, namely, for screening. Clearly, as we see coherent oscillations, the LLL, the interfering one, is not resistively connected to the OC. This crucial point is verified by measuring the current flowing into the OC, as detailed in Supplementary Note 7 . Measurement techniques Our electronic setup for measuring conductance and noise is detailed briefly in the Measurement Setup. We note that two amplifiers were utilized in the course of our measurements: the first, a homemade voltage preamplifier cooled to T =1 K having a gain factor 11 and a commercial amplifier (NF SA-220F5) at room temperature having a voltage gain 200. How to cite this article: Choi, H.K. et al. Robust electron pairing in the integer quantum hall effect regime. Nat. Commun. 6:7435 doi: 10.1038/ncomms8435 (2015).